Avalanche breakdown in GaTa4Se8−xTexnarrow-gap Mott insulators Mott transitions induced by strong electric fields are receiving growing interest. Recent theoretical proposals have focused on the Zener dielectric breakdown in Mott insulators. However, experimental studies are still too scarce to conclude about the mechanism. Here we report a study of the dielectric breakdown in the narrow-gap Mott insulators GaTa 4 Se 8− x Te x . We find that the I–V characteristics and the magnitude of the threshold electric field ( E th ) do not correspond to a Zener breakdown, but rather to an avalanche breakdown. E th increases as a power law of the Mott–Hubbard gap ( E g ), in surprising agreement with the universal law E th E g 2.5 reported for avalanche breakdown in semiconductors. However, the delay time for the avalanche that we observe in Mott insulators is over three orders of magnitude greater than in conventional semiconductors. Our results suggest that the electric field induces local insulator-to-metal Mott transitions that create conductive domains that grow to form filamentary paths across the sample. In many materials with partially filled d bands, electron motion is frozen as a result of strong repulsive interactions, which drive the system into a Mott insulating state [2] , [3] . Introduction of carriers in a Mott insulator often leads to exotic properties, such as high-Tc superconductivity in cuprates [4] and colossal magnetoresistance in manganites [5] . A Mott insulator can also be collapsed into a correlated metal by applying pressure. Notable examples are V 2 O 3 ( [6] ) and organics [7] . Another important type of Mott transition, which is receiving a great deal of attention, is the dielectric breakdown caused by strong electric fields. Many recent theoretical studies have focused on the Zener mechanism of breakdown for Mott insulators. For instance, calculations were performed in one-dimensional (1D) Hubbard chains using exact diagonalization [8] , [9] , [10] , [11] and time-dependent density matrix renormalization group [12] , or in the limit of large dimensions using dynamical mean field theory [13] . These theoretical studies predicted a similar non-linear behaviour in the current-voltage characteristics, and the existence of a threshold field ( E th ) beyond which a field-induced metal appears. In the latter case, where the Mott transition occurs beyond a critical value of the Coulomb interaction that is of similar magnitude as the bandwidth, it was found that E th is proportional to Δ 2 / v F , with Δ the charge gap, and v F the Fermi velocity. This implies a large threshold field of the order of 10 6 –10 7 V cm −1 , which is substantially larger than the experimental values observed in dielectric breakdown [14] . Surprisingly, compared with this significant theoretical effort, experimental studies of Mott insulators under strong electric fields remain quite scarce. Taguchi et al . [14] observed a dielectric breakdown in the quasi-1D Mott insulators Sr 2 CuO 3 and SrCuO 2 . More recently, a comparable dielectric breakdown was observed in the family of chalcogenide Mott insulators AM 4 Q 8 (A=Ga, Ge; M=V, Nb, Ta, Mo; Q=S, Se) [15] , [16] , [17] , [18] , [19] . However, in both cases, E th is of the order of 10 2 –10 4 V cm −1 , which does not match with theoretical predictions for Zener breakdown. This strong discrepancy therefore raises the question of the actual physical origin of the observed breakdown. Here we focus our study on the chalcogenide Mott insulators AM 4 Q 8 and show that the dielectric breakdown is consistent with an electric field-induced avalanche phenomenon rather than Zener breakdown. Our work reveals that the I ( V ) curve, the magnitude of E th and the dependence of E th versus the Mott–Hubbard gap are those expected for an avalanche breakdown, qualitatively similar to what is observed in semiconductors. However, our results also reveal significant differences, for instance, a delay time for the avalanche that is at least three orders of magnitude longer in the Mott insulators AM 4 Q 8 compared with the case of conventional band insulators. Mott–Hubbard gap evolution The lacunar spinel compounds AM 4 Q 8 , with tetrahedral transition metal clusters (see Fig. 1 ) [20] , represents an interesting family of narrow-gap Mott insulators. The low Mott gap value makes these compounds highly sensitive to doping or pressure. Doping of GaV 4 S 8 by Ti leads, for example, to a filling control insulator-to-metal transition (IMT) with the emergence of a ferromagnetic half metal [21] , [22] . On the other hand, an external pressure induces a bandwidth controlled IMT and superconductivity in GaTa 4 Se 8 [23] , [24] . Recently, we have reported that electric field leads to a striking volatile IMT or dielectric breakdown in GaTa 4 Se 8 [15] , [16] , [17] , [18] , which is qualitatively different from the non-volatile resistive switching based on electrochemical effects reported so far in many transition metal oxides [18] , [25] , [26] . 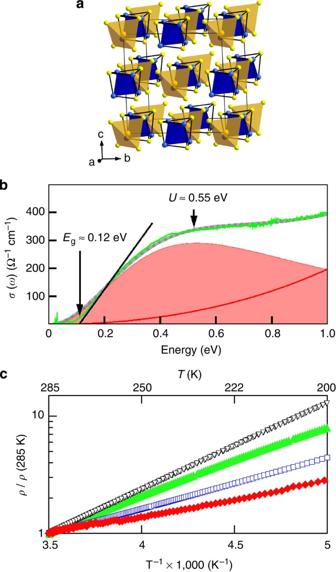Figure 1: Resistivity and optical conductivity measurements. (a) Representation of the lacunar spinel structure of the AM4Q8compounds. Blue-, orange- and yellow-filled circle represents M, A and Q atoms, respectively. The M4tetrahedral clusters and the AQ4tetrahedra are highlighted in blue and orange, respectively. (b) Experimental optical conductivity of GaTa4Se8(green line) showing that the optical conductivity is that expected for a Mott insulator with an Hubbard energyU=0.55 eV and a gap close to 0.12 eV. The grey solid line corresponds to the fit of optical conductivity spectrum using two contributions: a broad mid-infrared band (red shaded area) and high-frequencies contributions (thick solid red line). (c) Resistivity as a function of inverse temperature for GaTa4Se8(filled green triangle), GaTa4Se4Te4(black open triangle), GaTa4Se2Te6(blue open square) and GaTa4Se1.5Te6.5(filled red square). Figure 1: Resistivity and optical conductivity measurements. ( a ) Representation of the lacunar spinel structure of the AM 4 Q 8 compounds. Blue-, orange- and yellow-filled circle represents M, A and Q atoms, respectively. The M 4 tetrahedral clusters and the AQ 4 tetrahedra are highlighted in blue and orange, respectively. ( b ) Experimental optical conductivity of GaTa 4 Se 8 (green line) showing that the optical conductivity is that expected for a Mott insulator with an Hubbard energy U =0.55 eV and a gap close to 0.12 eV. The grey solid line corresponds to the fit of optical conductivity spectrum using two contributions: a broad mid-infrared band (red shaded area) and high-frequencies contributions (thick solid red line). ( c ) Resistivity as a function of inverse temperature for GaTa 4 Se 8 (filled green triangle), GaTa 4 Se 4 Te 4 (black open triangle), GaTa 4 Se 2 Te 6 (blue open square) and GaTa 4 Se 1.5 Te 6.5 (filled red square). Full size image To study the origin of this dielectric breakdown and to explore its relationship with the Mott–Hubbard gap, we have investigated the electric field effects in the series of compounds GaTa 4 Se 8− x Te x ( x =0, 4.0, 6.0 and 6.5). These compounds were synthesized as described elsewhere [27] . Optical conductivity and resistivity measurements were subsequently undertaken to evaluate the gap evolution in this series. The room temperature optical conductivity of GaTa 4 Se 8 , shown in Fig. 1b , displays all the expected features of a narrow-gap Mott Insulator with a Hubbard energy ( U ) of the order of 0.55 eV [28] . The low-bias resistivities ρ ( T ) measured with a standard four-probe technique for the series of compounds GaTa 4 Se 8− x Te x exhibit a semiconducting-like behaviour with a temperature dependence consistent with an activation law at high temperature (see Fig. 1c ). The systematic change of the activation energy observed in Fig. 1 suggests that the substitution of Se per Te permits the bandwidth control of the Mott–Hubbard gap (from 100 to 300 meV) within the GaTa 4 Se 8− x Te x series of compounds, thus enabling the study of the threshold field dependence with the size of the gap. Dielectric breakdown experiments Dielectric breakdown was systematically studied in this series of narrow-gap Mott insulators using a procedure described in the Methods section. 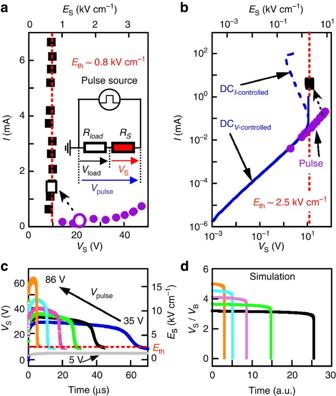Figure 2: Resistive switching experiments and modelling. (a)I–Vcurves extracted from pulse (open circles and squares) experiments for a crystal of GaTa4Se1.5Te6.5. The circuit used to apply voltage pulses is shown in inset. (b)I–Vcurves extracted from pulse (open circles and squares) or DC experiments (plain or dashed lines) for a crystal of GaTa4Se8. (c) Evolution of the voltageVS(t) across a crystal of GaTa4Se8when short voltage pulsesVpulse(10–70 μs) of increasing magnitude are applied to the circuit. For example,Vpulse=5, 35, 40, 44, 50, 60 and 86 V for the grey, blue, black, green, pink, light blue and orange curves, respectively. These curves show a clear evolution of the time (tdelay) at which the transition to a low resistance state (resistive switching) occurs as a function ofVpulse. Inaandb, theI–Vcurves are extracted fromVS(t) curves similar to the one shown incand from the correspondingI(t) curves not shown here. Inaandb, open circles correspond to theI–Vvalues measured before the resistive switching, and open squares correspond to theI–Vvalues measured after the resistive switching. (d) Results of mathematical modelling ofVS(t) using a 1D resistive network. The time at which the resistive switching occurs decreases as the applied voltage to the resistor network is increased from the black to the orange curve. Figure 2 shows that these compounds undergo a sudden volatile dielectric breakdown above a certain threshold electric field (≈1–10 kV cm −1 ). As an example, Fig. 2c depicts the typical temporal evolution of the voltage V s ( t ) across a GaTa 4 Se 8 crystal while a series of short (10–70 μs) voltage pulses ( V pulse ) are applied. When the electric field applied to the crystal exceeds a threshold field of ≈2.5 kV cm −1 , the crystal systematically undergoes a fast transition to a low resistance state (that is, from 70 to 5 kΩ) called a dielectric breakdown or resistive switching. This transition is volatile and perfectly reproducible. In fact, after the pulse application, the low-bias resistance returns to its original value. The delay t delay between the application of the pulse and the dielectric breakdown shifts to smaller values with increasing applied voltage. The voltage drop on the sample V S in the breakdown state is always V S ≈9 V (or E S ≈2.5 kV cm −1 ) whatever the voltage applied to the sample before the resistive switching. On the other hand, the current flowing through the sample after the dielectric breakdown shows a highly non-ohmic behaviour in the transited state in both, pulse or dc measurements (see Fig. 2b ). Thus, we infer that E th (that is, V th / d where d is the distance between electrodes) corresponds to the breakdown field for the limiting case t delay → ∞ . The same qualitative behaviour was observed for GaTa 4 Se 1.5 Te 6.5 (see Fig. 2a ), all other GaTa 4 Se 8− x Te x compounds and more generally for all AM 4 Q 8 (A=Ga, Ge; M=V, Nb, Ta, Mo; Q=S, Se) Mott-insulator compounds [18] . Figure 2: Resistive switching experiments and modelling. ( a ) I–V curves extracted from pulse (open circles and squares) experiments for a crystal of GaTa 4 Se 1.5 Te 6.5 . The circuit used to apply voltage pulses is shown in inset. ( b ) I–V curves extracted from pulse (open circles and squares) or DC experiments (plain or dashed lines) for a crystal of GaTa 4 Se 8 . ( c ) Evolution of the voltage V S ( t ) across a crystal of GaTa 4 Se 8 when short voltage pulses V pulse (10–70 μs) of increasing magnitude are applied to the circuit. For example, V pulse =5, 35, 40, 44, 50, 60 and 86 V for the grey, blue, black, green, pink, light blue and orange curves, respectively. These curves show a clear evolution of the time ( t delay ) at which the transition to a low resistance state (resistive switching) occurs as a function of V pulse . In a and b , the I–V curves are extracted from V S ( t ) curves similar to the one shown in c and from the corresponding I ( t ) curves not shown here. In a and b , open circles correspond to the I–V values measured before the resistive switching, and open squares correspond to the I–V values measured after the resistive switching. ( d ) Results of mathematical modelling of V S ( t ) using a 1D resistive network. The time at which the resistive switching occurs decreases as the applied voltage to the resistor network is increased from the black to the orange curve. Full size image Dielectric breakdown mechanism For conventional semiconductors, the dielectric breakdown is well documented and different mechanisms are proposed such as Zener tunnelling [29] or avalanche process [30] . The threshold field observed in the AM 4 Q 8 compounds is at least three orders of magnitude smaller than the threshold field of the order of 10 6 –10 7 V cm −1 expected for Zener breakdown in Mott insulators [8] . This definitively rules out a Zener breakdown mechanism. Conversely, the magnitude of the threshold field in AM 4 Q 8 Mott insulators compares well with the threshold field values of 1 and 40 kV cm −1 observed for avalanche breakdowns in narrow-gap semiconductors InSb and InAs, respectively [31] , [32] . The I ( V ) characteristics observed in the AM 4 Q 8 compounds and in semiconductors like InSb, InAs, Si or Ge are also very similar [30] . Indeed, all these compounds exhibit a steep increase of the current at the threshold field, which is almost vertical. In narrow-gap semiconductors, this is related to the impact-ionization process. An avalanche breakdown indeed occurs when the electrons accelerated by the applied voltage can gain enough energy to ionize by impact of other electrons above the band gap and generate electron-hole pairs [30] . When the creation of electron-hole pairs by impact-ionization overcompensates the electron-hole recombination process (Auger Thermal process), a multiplication of carriers occurs and induces a dielectric breakdown with a steep increase of the current at the threshold field. For high current density, the avalanche breakdown is characterized by a negative differential resistance in the current-voltage characteristic, which is the consequence of the contribution of holes to the field distribution along the sample [30] . As shown in Fig. 2 , such a negative differential resistance effect is observed on the I–V curve of GaTa 4 Se 8 measured in DC mode using a current source. Again, this strongly supports an avalanche mechanism as the origin of the dielectric breakdown. Dependence of the avalanche threshold field For semiconductors, the avalanche threshold field varies as a function of a power law of the band gap [30] and follows the universal law E th E g 2.5 ( [31] , [32] ). For comparison, Fig. 3 displays the variation of the threshold field as a function of the Mott–Hubbard gap for all the AM 4 Q 8 compounds. This figure reveals a remarkable power law dependence of the threshold fields with the gap E th E g 2.5 (see blue curve in Fig. 3 ). The inset of Fig. 3 also compares the threshold fields versus gap dependence for the AM 4 Q 8 compounds and classical semiconductors. This comparison reveals that for all Mott and band insulators or semiconductors, the threshold fields line up along a universal law E th E g 2.5 . This is again strong evidence that the breakdown observed in the Mott insulators AM 4 Q 8 originates from an avalanche phenomenon. 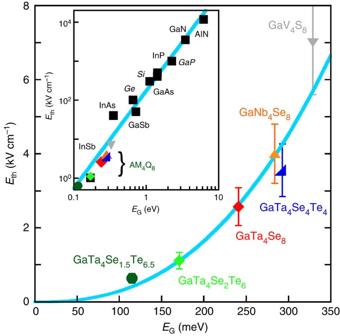Figure 3: Dependence ofEthin Mott insulators and semiconductors. Threshold electric field (inducing avalanche breakdown) as a function of the Mott gap for various AM4Q8compounds. The solid blue curve correspond to a power law dependenceEthEg2.5. Inset: comparison of the threshold fields versus gap dependence for the AM4Q8compounds and for classical semiconductors. The solid blue line displays the universal lawEth(kV cm−1)=173Eg(eV)2.5observed for semiconductors. Figure 3: Dependence of E th in Mott insulators and semiconductors. Threshold electric field (inducing avalanche breakdown) as a function of the Mott gap for various AM 4 Q 8 compounds. The solid blue curve correspond to a power law dependence E th E g 2.5 . Inset: comparison of the threshold fields versus gap dependence for the AM 4 Q 8 compounds and for classical semiconductors. The solid blue line displays the universal law E th (kV cm −1 )=173 E g (eV) 2.5 observed for semiconductors. Full size image This scaling of Mott- and band-insulators along the same universal law, E th =1.73 E g 2.5 , indicates that the threshold field in the avalanche breakdown depends only on the gap whatever its origin and nature. This is rather surprising as the excitation gap in Mott insulators arises from electron–electron repulsions (that is, from strong correlation effects), in stark contrast with the case of conventional semiconductors. Despite this similarity, as we mentioned before, the main qualitative difference between the electric breakdown in semiconductors and Mott insulators is the significantly longer t delay of the latter. The origin of the difference may be due to the different coupling to the lattice degrees of freedom. The Mott transition is indeed accompanied of a compressibility anomaly [33] , [34] , which leads to a large volume change [35] . In fact, the giant electromechanical coupling observed during an STM studies by applying electric pulses between the tip and a cleaved GaTa 4 Se 8 crystal surface supports this scenario [17] . Therefore, the strong coupling of the electronic and lattice degrees of freedom is likely to slow down significantly the velocity of the avalanche propagation. Interestingly, Fig. 2 shows that the dielectric breakdown in the AM 4 Q 8 Mott insulators occurs with a t delay in the μs range (from a few μs to the ms) for typical sample lengths d =20–40 μm. In contrast, in semiconductors, the t delay lies in the ps to the ns range, that is, several orders of magnitude faster [30] . 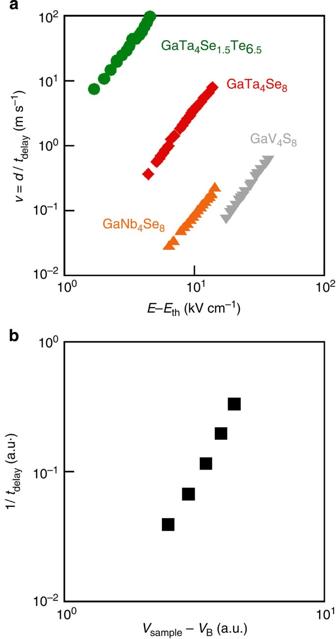Figure 4: Avalanche velocity in Mott insulators. (a) Avalanche velocityv=d/tdelayfor various AM4Q8compounds as a function of excess electric fieldE–EthwhereEis the electric field applied on the sample. (b) Velocity of the transition 1/tdelayextracted from the mathematical modelling of the resistive switching shown inFig. 2d. Figure 4 displays the avalanche velocity v = d / t delay as a function of excess electric field E–E th where E is the electric field applied on the sample. This figure shows that v varies as ( E–E th ) 3 . This remarkable power law dependence as well as the magnitude of the velocity in m s −1 range recall a phase growth mechanism [36] or the propagation of dislocations [37] , [37] . This analysis therefore suggests that the excess electric field triggers the local growth of conducting domains where a Mott transition has taken place, which eventually form filamentary paths across the sample as the avalanche breakdown occurs. Figure 4: Avalanche velocity in Mott insulators. ( a ) Avalanche velocity v = d / t delay for various AM 4 Q 8 compounds as a function of excess electric field E – E th where E is the electric field applied on the sample. ( b ) Velocity of the transition 1/ t delay extracted from the mathematical modelling of the resistive switching shown in Fig. 2d . Full size image A mathematical modelling of the previous scenario was undertaken to describe the experimental data. This model considers a 1D resistive network where each cell may be in one of two states, insulator (I) or metal (M), characterized by their corresponding resistance r I and r M , and their energy E I and E M , respectively. This model also assumes that the two states are separated by an energy barrier of height E B − E I . The energy landscape used for the calculation is shown in Supplementary Fig. S1 . Initially, all cells are in the insulating state, because the system is a Mott insulator. An external voltage pulse V pulse is then applied on the resistor network, and the local voltage drops on the cells are computed. The cells may undergo a transition from state I to M by a thermal activation process. The effective activation energy barrier, for an IMT of the i th cell under the action of the applied voltage, is E B – E I –ΔV i , where ΔV i is the computed voltage drop at the cell. These assumptions lead to non-linear differential equation for the rate of cell transitions per unit time. Further details of the mathematical expressions are provided in the Methods section. The solution of the differential equation is easily obtained by standard numerical integration. The results are shown in Fig. 2d . We observe that this simple model qualitatively captures the behaviour of t delay of the avalanche mechanism. Initially, the conductive path modelled by the resistive network is highly resistive, so there is a small voltage drop on each cell, and the rate of transitions is low. Successive transitions, however, lower the resistance of the path, as r M << r I , therefore increasing the current and also the voltage drop ΔV i in the cells that still remain insulating. The increased ΔV i lowers the local energy-activation barriers, thus augmenting the transition rates. A larger fraction of cells undergo a transition and, eventually, a runaway process takes place where the rest of the cells rapidly completes their transitions. Interestingly, this simple model also qualitatively accounts for the field dependence of the velocity of the transition as shown in Supplementary Fig S2 and in Fig. 4 . However, the power law behaviour predicted by this simple model is parameter dependent, that is, is non universal. To conclude, we have reported for the first time an avalanche breakdown in the narrow-gap Mott insulators AM 4 Q 8 . The phenomenology of the breakdown ( I ( V ) characteristic) and the magnitude of the threshold electric field are comparable with those reported for avalanche breakdowns in semiconductors. Moreover, the threshold field dependence with the width of the Mott–Hubbard gap shows a surprising agreement with the universal law E th =1.73 E g 2.5 reported for semiconductors, despite the fact that the AM 4 Q 8 are strongly correlated systems. Our experimental and theoretical investigations suggest that, unlike semiconductors, avalanche breakdown in Mott insulators is associated with the growth of conducting filamentary paths of a metallic metastable phase within the sample. The strong coupling of electronic and lattice degrees of freedom due to compressibility anomalies may account for the reduced avalanche speed observed in the Mott insulators compared with conventional band insulators. Finally, our work suggests that avalanche breakdown may be a general feature of narrow-gap Mott insulators. Sample preparation Single crystals of GaTa 4 Se 8− y Te y with y ranging from 0 to 6.5 were prepared using stoichiometric mixtures of elemental gallium, tantalum, selenium and tellurium (purities ≥99.5 %) ( [27] ). These mixtures were loaded in evacuated sealed quartz ampules of about 10 cm and heated up at 300 °C h −1 to 1,000 °C and hold at this temperature during 160 h. The quartz tubes were subsequently cooled down, first slowly to 800 °C at 1 °C h −1 and then faster (300 °C h −1 ) to room temperature. These syntheses yielded black powders containing a high yield of GaTa 4 Se 8− y Te y metallic grey cubic and tetrahedral crystals (typical size ≤300 μm) along with a small amount of impurity phases (for example, GaTe and TaSe 2 ). Large amounts of tetrahedral or cubic-shaped crystals of all other members of the AM 4 Q 8 family have been obtained using a similar procedure. Transport measurements The AM 4 Q 8 crystals used for transport measurements were contacted using 17 μm gold wires and carbon paste (Electrodag PR-406), and then annealed in vacuum at 150 °C during 30 min. The low-bias resistance of the AM 4 Q 8 was measured using a source-measure unit (either a Keithley 236 or a Keithley 6430) by a standard two- or four-probe technique. We checked that the contact resistances were much smaller than the sample resistance. Voltage pulses were applied using an Agilent 8114A. During the pulse, the voltage and current across the sample were measured with a Tektronix DPO3034 oscilloscope associated with a IeS-ISSD210 differential probe, using the simple circuit described in the inset of Fig. 2a . Mathematical modelling To obtain Figs 2d and 4b , we numerically integrated by using fourth-order Runge–Kutta method (time step=0.001). Here x is the fraction of cells in metallic state. V B is defined as the voltage that cancels the energy barrier ( E B − E I ) in all cells when x =0. E B , E I and ΔV i are defined as displayed in Supplementary Fig. S1 . We set ν =0.001, k B T =1, E B − E I =1 and For Fig. 2d , we simulated V pulse =2.5, 3, 3.5, 4, 4.5, 5 and 5.5. Figure 4b presents the switching times for the five higher values. The 1D resistivities were set as 10 · r M = R L and r I =10 · R L . V S was obtained as: was calculated as the inverse of the number of Runge–Kutta cycles needed for x to arrive to 1. Another output of this numerical simulation is presented in Supplementary Fig. S2 , the evolution of in time. How to cite this article: Guiot, V. et al . Avalanche breakdown in GaTa 4 Se 8− x Te x narrow-gap Mott Insulators. Nat. Commun. 4:1722 doi: 10.1038/ncomms2735 (2013).